Runx-dependent and silencer-independent repression of a maturation enhancer in theCd4gene An intronic silencer, S4 , in the Cd4 gene has been shown to be responsible for the helper-lineage-specific expression of CD4; S4 requires Runx complex binding to exert its silencer function against the enhancer-mediated Cd4 activation by modulating the epigenetic state of the Cd4 gene. Here we identify a late-acting maturation enhancer. Bcl11b plays essential roles for activation of both the early-acting proximal enhancer and maturation enhancer of Cd4 . Notably, Runx complexes suppress these enhancers by distinct mechanisms. Whereas repression of the proximal enhancer depends on the S4 silencer, the maturation enhancer is repressed by Runx in the absence of S4 . Moreover, ThPOK, known to antagonize S4 -mediated Cd4 repression, assists Runx complexes to restrain maturation enhancer activation. Distinct modes of S4 silencer action upon distinct enhancers thus unravel a pathway that restricts CD4 expression to helper-lineage cells by silencer-independent and Runx-dependent repression of maturation enhancer activity in cytotoxic-lineage cells. CD4 and CD8 glycoproteins function as a co-receptor that assists T-cell antigen receptor (TCR) to recognize antigenic peptide presented by major histocompatibility complex (MHC) class II and class I molecules, respectively [1] . In addition, CD4/CD8 molecules serve as useful markers to define thymocyte developmental stages and helper-lineage and cytotoxic-lineage T cells [2] . Signals from pre-TCR complexes in CD4 − CD8 − double-negative (DN) thymocyte progenitors induce both CD4 and CD8 expression, resulting in the generation of CD4 + CD8 + double-positive (DP) precursor thymocytes. A limited numbers of DP thymocytes, which have passed a process known as positive selection, differentiate further into mature thymocytes [3] . Post-selection thymocytes expressing MHC-class I (MHC-I) restricted TCRs are specified to differentiate into the cytotoxic-lineage and acquire CD4 − CD8 + single-positive (SP) phenotype by terminating CD4 expression, whereas MHC-class II (MHC-II)-mediated TCR engagement generates CD4 + CD8 − SP thymocytes committed to the helper-lineage by inhibiting CD8 expression. Such stage-specific and lineage-specific expression of CD4/CD8 co-receptors is regulated at the transcriptional level by a combinational regulation of cis -regulatory elements [2] . For instance, insertion of a 434 bp intronic transcriptional silencer ( S4 ) into a transgene together with a 430 bp proximal enhancer ( E4p ) and a minimal Cd4 promoter ( P4) is necessary to recapitulate stage-specific and lineage-specific Cd4 expression in reporter transgene expression [4] , [5] . CD4 de-repression from CD8 + T cells upon ablation of the S4 sequences [6] , [7] . These observations established a model that the single S4 silencer controls helper-lineage specific expression of the Cd4 gene [8] . Sequential studies further revealed that binding of Runx transcription factor complexes to S4 through their recognition of two Runx-motifs is essential for S4 activity [9] , [10] . Ablation of the E4p from the murine Cd4 locus ( Cd4 ΔE4p/ΔE4p mice) also confirmed that E4p is essential to initiate Cd4 activation [11] . However, despite severely diminished CD4 expression on precursor thymocytes, a small but significant proportion of precursors was positively selected and differentiated into mature thymocytes expressing CD4 at a lower level in Cd4 ΔE4p/ΔE4p mice, leading to an assumption that additional enhancer(s), referred to as a maturation enhancer ( E4m ), should be present [11] . It has also been shown that stage-specific DNA de-methylation in helper-lineage cells and continuous DNA methylation in cytotoxic-lineage cells are involved in establishment of the heritable active and silent status, and requires E4p and S4 activity, respectively [11] , [12] . Thus, Cd4 gene regulation has served as an ideal model to study how stage-specific and lineage-specific epigenetic modifications are regulated by cis -regulatory elements. However, the genomic region containing E4m activity remains elusive, as does the mechanism by which E4m activity is regulated. In this study, we identify the E4m , validated its role in regulating CD4 expression, and isolate Bcl11b as an important activator for E4m . We also show that Runx complexes repress the E4m activity in CD8 + T cells even in the absence of the S4 and find unexpected ThPOK function that prevents premature E4m activation by assisting Runx-mediated E4m repression. Collectively, our results reveal that Runx complexes repress two enhancers, E4p and E4m , in distinct manners, providing a novel insight that revises a silencer-based model for a lineage-specific Cd4 expression. Rescue of E4p function by a heterologous enhancer It was shown that E4p is necessary for DNA de-methylation of the Cd4 gene [12] . To examine whether the activity that induces DNA de-methylation in the Cd4 locus is specific to E4p , we tested how a heterologous enhancer behaves in the Cd4 locus. Two enhancers, a thymic enhancer ( TE ) and a proximal enhancer ( PE ), are present in the Thpok gene encoding the CD4-specific transcription factor ThPOK [13] , [14] . Low expression of Thpok upon removal of Tet family proteins that are essential for DNA de-methylation [15] suggests an involvement of DNA de-methylation in activation of the Thpok gene. In order to replace E4p sequence in the Cd4 locus with the two separately located enhancers in the Thpok locus, we synthesized an Eth DNA fragment in which core sequences of TE and PE were conjugated (Supplementary Fig. 1a ), and generated a Cd4 Eth allele through homologous recombination in embryonic stem (ES) cells (Fig. 1a and Supplementary Fig. 1b ). Fig. 1 Enhancer replacement between Cd4 and Thpok genes. a Schematic structures of mutant Cd4 alleles. Ovals marked with different colors represent c is -regulatory regions, Cd4 silencer ( S4 ), Cd4 proximal enhancer ( E4p ), and synthetic Thpok enhancer ( Eth ). The black box and triangle represent exons and loxP sequences, respectively. b Dot plots showing CD4 and CD8 expression and histograms at the right showing CD4 expression in indicated cell subsets from mice with indicated genotypes. Numbers in quadrants indicate respective cell percentage. Representative results of at least three independent analyses. c Graph showing relative Cd4 to Hprt mRNA in pre-selection CD24 hi TCRβ lo thymocytes, CD24 lo TCRβ hi CD4 single positive (SP), and CD24 lo TCRβ hi CD8 SP thymocytes of mice with indicated genotypes. Means ± SD. *** p < 0.001, * p < 0.05 ((One-way ANOVA and Tukey’s multiple comparison test)). d Pseudocolor plots showing CD4 expression and cell divisions five days after in vitro stimulation of sorted CD4 + T cells from mice with indicated genotype. Numbers in the indicated gate represent cell percentages. e Bisulfite PCR at six amplicons from the first intron in the Cd4 gene in naïve CD4 + T cells from mice with indicated genotypes. Symbols indicate methylated (black filled circle) or un-methylated (black open circle) CpG motifs. The lower graph shows the summary of three independent experiments. Means ± SD. *** p < 0.01 (unpaired student t test, two-sided) Full size image CD4 expression on Cd4 Eth/Eth thymocytes at the DP stage, defined as the CD24 hi TCRβ lo population, was lower than that in control Cd4 +/+ but higher than that in Cd4 ΔE4p/ΔE4p cells (Fig. 1b, c ). Given that the activity of TE and PE in the Thpok locus was low in pre-selection DP thymocytes and gradually increased during thymocytes maturation [13] , [14] , [16] , Eth activity in the Cd4 locus was likely to retain original stage-specificity and not be sufficient to completely restore CD4 expression in precursor DP thymocytes. However, during maturation into the helper-lineage, the CD4 expression level from the Cd4 Eth allele closely approached that from the wild-type Cd4 allele (Fig. 1b, c , and Supplementary Fig. 1c ). We next examined whether CD4 expression from the Cd4 Eth allele could be stably maintained after cell division. Although the CD4 expression level from the Cd4 ΔE4p allele was decreased according to the rounds of cell divisions as previously reported [11] , [12] , CD4 expression was retained at a higher level in CD4 + cells from Cd4 Eth/Eth mice (Fig. 1d ). DNA de-methylation at the intronic region was induced in Cd4 Eth/Eth cells to a similar extent as that in control Cd4 +/+ cells, whereas DNA remained significantly methylated in Cd4 ΔE4p/ΔE4p cells (Fig. 1e ). These observations indicated that the synthetic heterologous Eth enhancer was able to restore E4p function in the Cd4 locus to a degree sufficient to establish a heritable actives state at least in part through the induction of DNA de-methylation. Characterization of the Cd4 maturation enhancer ( E4m ) In the murine Cd4 locus, the presence of a Cd4 maturation enhancer ( E4m ) shortly downstream of S4 has been predicted [17] . We found conserved sequences at approximately 1 kb downstream of the S4 region (Supplementary Fig. 2a ); moreover, the public ATAC-Seq database showed that this region become more accessible specifically in CD4-lineage cells after positive selection, whereas the S4 region became more accessible in CD8-lineage cells (Supplementary Fig. 2a ). In addition, our chromatin immunoprecipitation (ChIP) combined with sequencing (ChIP-Seq) analysis detected binding of Runx complexes to S4 and its downstream region in total thymocytes (Fig. 2a ). Furthermore, changes of post-translational modifications on K27 of histone 3 for tri-methylation (H3K27me3) and for acetylation (H3K27ac), which are known as markers for inactive and active enhancer states [18] , respectively, indicated that H3K27ac at E4p was highest in precursor DP thymocytes, whereas H3K27ac was increased at a the putative E4m region in post-selection (CD69 + CD24 hi TCRβ + ) thymocytes. In comparison, H3K27me3 modification accumulated at both regions specifically in CD8 + T cells. Together, these features prompted us to test the function of this putative E4m region genetically by deleting the 337 bp core conserved sequences. Accordingly, by using an ES cell clone harboring a Cd4 +/+ or Cd ΔS4/ΔE4p genotype (Supplementary Fig. 2b, c ), we established two mouse lines harboring Cd4 ΔE4m and Cd4 ΔE4p:ΔE4m alleles, with the latter lacking both E4p and E4m (Supplementary Fig. 2b, c ). Strikingly, CD4 expression during T cell development was completely abolished in the Cd4 ΔE4p:ΔE4m/ΔE4p:ΔE4m mice (Fig. 2b ). This finding demonstrated not only that enhancer activity complementing CD4 expression ( E4m ) from the Cd4 ΔE4p allele is embedded on the deleted region, but also that E4p and E4m serve as major enhancers to drive CD4 expression in T cells. Fig. 2 Effects of loss of the maturation enhancer, E4m , on CD4 expression. a Upper graphs showing kinetic changes of H3K27ac and H3K27me3 at E4p and E4m regions in pre-selection (DP), freshly selected (CD69 + ), and CD4 SP (4SP) and CD8 SP (8SP) thymocytes. Summary of three independent ChIP experiments. Means ± SD. (Middle) Runx ChIP-Seq track at the Cd4 gene in total thymocytes. Gene structures and regulatory regions are shown as in Fig. 1a . Schematic structures of mutant Cd4 alleles are shown at the bottom. b Pseudocolor plots showing CD4 and CD8 expression in indicated cell subsets from mice with indicated genotypes. Numbers in quadrants indicate respective cell percentages. Representative results of at least three independent analyses of each genotype. c Histograms showing CD4 expression levels on CD24 hi TCRβ lo , CD8-negative CD24 hi TCRβ hi and CD8-negative CD24 lo TCRβ hi thymocytes from Cd4 +/+ (dotted), Cd4 ΔE4p/ΔE4p (red), and Cd4 ΔE4m/ΔE4m (green) mice. One representative of three analyses. d Pseudocolor plots showing CD4 expression and cell divisions five days after in vitro stimulation of sorted peripheral CD4 + T cells from mice with indicated genotypes. Numbers in the indicated gate represent cell percentages. e Bisulfite PCR analyses of naïve CD4 + T cells from Cd4 +/+ and Cd4 ΔE4m/ΔE4m mice are shown as in Fig. 1d . The right graph shows a summary of three independent experiments. Means ± SD. ** p < 0.01 (unpaired student t test, two-sided). f Graph showing percentage of CD4 + CD8 − cells in mature (CD24 lo TCRβ hi ) thymocytes and the lymph node TCRβ + population of Cd4 +/+ and Cd4 ΔE4m/ΔE4m mice. Means ± SD. *** p < 0.001 (unpaired student t test, two-sided) Full size image We next examined the impact of the E4m deletion alone on CD4 expression and T cell development in Cd4 ΔE4m/ΔE4m mice. Although the CD4 expression level at the DP stage was compatible between Cd4 +/+ and Cd4 ΔE4m/ΔE4m cells, it became lower in Cd4 ΔE4m/ΔE4m cells than that in Cd4 +/+ cells at the CD8 − CD24 hi TCRβ hi stage (Fig. 2b, c ). Notably, CD4 expression level from the Cd4 ΔE4p allele was higher than that from the Cd4 ΔE4m allele in CD8 − CD24 hi TCRβ hi cells, although CD4 expression levels from these two mutant Cd4 alleles became similar to each other and lower than that from the wild-type Cd4 allele in mature (CD24 lo TCRβ hi ) CD8 − thymocytes. Thus, the Cd4 ΔE4p allele could induce CD4 expression faster than the Cd4 ΔE4m allele after positive selection, although changes of histone modification patterns at the E4p was equivalent between control Cd4 and Cd4 Δ E4m alleles ( Supplementary Fig. 3 ). Following activation of CD4 + CD8 − splenic T cells, CD4 expression from the Cd4 ΔE4m allele decreased to a similar extent as that from the Cd4 ΔLS allele (Fig. 2d ), in which both S4 and E4m were deleted [6] . However, the percentage of cells retaining CD4 expression was higher in Cd4 ΔE4m/ΔE4m cells than in Cd4 ΔE4p/ΔE4p cells, although the percentage of methylated CpG motifs at intronic regions remained higher in these two cell types to a similar extent (Figs 1c and 2e ). These results indicated that E4m activity is also necessary to establish a heritable active state at the Cd4 locus in part by activating the DNA de-methylation process together with E4p . Of note, a percentage of CD4 + CD8 − cells among the mature thymocyte and lymph node T cell population was decreased in Cd4 ΔE4m/ΔE4m mice (Fig. 2b, f ). To examine whether re-directed differentiation of MHC-II selected cells was involved in the decrease of CD4 + T cells, as was observed in Cd4 ΔE4p/ΔE4p mice [11] , we analyzed the differentiation of MHC-II selected cells under β2-microglobulin-deficient condition. In CD24 lo TCRβ hi thymocyte population, while CD4 − CD8 + cells were undetectable in control B2m −/− : Cd4 +/+ mice, mature CD4 − CD8 + SP thymocytes emerged in B2m −/− : Cd4 ΔE4m/ΔE4m mice (Fig. 3a, b ). In the CD24 hi TCRb hi population, the percentages of CD8 expressing cells were also higher in B2m −/− : Cd4 ΔE4m/ΔE4m mice (Fig. 3a ). As ThPOK is involved in terminating CD8 expression during the maturation of MHC-II selected cells [19] , [20] , we analyzed Thpok expression using the Thpok gfp reporter allele [16] . Although the majority of MHC-II selected CD24 hi TCRb hi thymocytes in B2m −/− : Cd4 +/+ mice expressed Thpok-gfp at a higher level, biphasic and lower Thpok-gfp expression was observed in those cells in B2m −/− : Cd4 ΔE4m/ΔE4m mice (Fig. 3c ), and the CD8 expression level remained higher in Thpok-gfp lo cells than in Thpok-gfp hi cells (Fig. 3c ). These observations suggested that a low and delayed CD4 expression after positive selection in the absence of E4m resulted in a re-direction of some MHC-II selected thymocytes to the CD8-lineage in part through impaired Thpok induction. Fig. 3 Re-directed differentiation of MHC-II selected thymocyte by loss of the E4m enhancer. a , b Dot plots in a showing CD4 and CD8 expression in indicated cell subsets from B2m −/− : Cd4 +/+ and B2m −/− : Cd4 ΔE4m/ΔE4m mice. Graphs in b showing summary of percentage of CD4 − CD8 + cells in mature (CD24 lo TCRβ hi ) thymocytes and the lymph node (LN) TCRβ + population. Means ± SD. ** p < 0.01, *** p < 0.001 (unpaired student t test, two-sided). c Histogram at left showing Thpok-gfp expression in freshly-selected (CD24 hi TCRβ hi ) thymocytes of B2m −/− : Cd4 +/+ and B2m −/− : Cd4 ΔE4m/ΔE4m mice. Histogram at right showing CD8 expression in Thpok-gfp lo and Thpok-gfp hi CD24 hi TCRβ hi thymocytes of B2m −/− : Cd4 ΔE4m/ΔE4m mice. One representative result of two mice. d Dot plots showing CD4 and CD8 expression three and five days after TCR stimulation of sorted CD4 − CD8 + mature thymocytes from B2m +/− : Cd4 +/ΔE4m and B2m −/− : Cd4 ΔE4m/ΔE4m mice. Numbers in quadrants indicate respective cell percentages. e IL7R expression in CD4 − CD8 + thymocytes (left) and phosphorylated Stat5 levels in CD4 − CD8 + thymocytes (right) at 5 and 15 min following IL7 stimulation at indicated concentrations from B2m +/− : Cd4 +/ΔE4m and B2m −/− : Cd4 ΔE4m/ΔE4m mice are shown. Numbers in left histograms indicate mean fluorescence intensity (MFI) Full size image However, the percentage of CD4 − CD8 + subset cells declined in the peripheral lymphoid tissues of B2m −/− : Cd4 ΔE4m/ΔE4m mice (Fig. 3b ). This might be explained by the differentiation of CD4 − CD8 + thymocytes into CD4 + CD8 − T cells or a defect in the survival of CD4 − CD8 + thymocytes in those mice. To trace CD4 and CD8 expression, we cultured CD4 − CD8 + thymocytes prepared from B2m −/− : Cd4 ΔE4m/ΔE4m mice and found that these cells remained as CD4 − CD8 + cells after five days (Fig. 3d ). It has been shown that IL-7 signaling is crucial for the survival and expansion of CD8 SP thymocytes [21] , [22] . Consistent with a lower IL-7R expression level in the CD4 − CD8 + thymocytes of B2m −/− : Cd4 ΔE4m/ΔE4m mice than in control MHC-I restricted CD4 − CD8 + thymocytes (Fig. 3e ), the phosphorylation of Stat5 after in vitro IL-7 stimulation was reduced in B2m −/− : Cd4 ΔE4m/ΔE4m CD4 − CD8 + thymocytes (Fig. 3e ). These results suggested that the low level of IL-7R expression in re-directed CD4 − CD8 + thymocytes is involved in the decline in the percentage of CD4 − CD8 + subset in the periphery of B2m −/− : Cd4 ΔE4m/ΔE4m mice. Bcl11b is essential for activation of E4p and E4m enhancers To understand how E4m function is regulated, it is necessary to identify molecules that bind and regulate E4m activity. During analyses of Bcl11b function [23] , we observed that Bcl11b associates with the E4p , S4 , and E4m regions in total thymocytes (Fig. 4a ). ChIP-qPCR showed that associations of both Runx and Bcl11b with the E4p were dramatically decreased in peripheral T cells (Fig. 4b ). Runx binding to S4 was the highest in CD8 + T cells but was almost lost in CD4 + T cells, with Bcl11b binding to S4 also becoming lower in CD4 + T cells compared to that in other cell subsets (Fig. 4b ). Although the association of Runx to E4m was compatible between the three cell subsets, Bcl11b binding to E4m was higher in CD4 + T cells than in CD8 + T cells (Fig. 4b ). Fig. 4 Requirement for Bcl11b in activating Cd4 at two stages. a ChIP-Seq tracks at the Cd4 gene showing binding of Bcl11b in total thymocytes. b ChIP-qPCR analyses for Runx (left) and Bcl11b (right) bindings to the Cd4 proximal enhancer ( E4p ), Cd4 silencer ( S4 ), and Cd4 maturation enhancer ( E4m ) in DP thymocytes, peripheral CD4 + ,and CD8 + T cells. N.C.: negative control region. Summary of three independent ChIP experiments. Means ± SD. * p < 0.05 (One-way ANOVA and Tukey’s multiple comparison test). c Contour plots showing CD4 and CD8 expression in indicated thymocyte subsets of Bcl11b +/+ and Bcl11b m/m newborn mice. Numbers in quadrants indicate respective cell percentages. Representative results of at least three independent analyses. d Summary of percentage of indicated cell types in indicated cell populations of Bcl11b +/+ and Bcl11b m/m mice. Means ± SD. *** p < 0.001 (unpaired student t test, two-sided). e Contour plots showing CD4 and CD8 expression in indicated thymocyte subsets and lymph node (LN) T cells of mice with indicated genotypes. Numbers in quadrants indicate respective cell percentages. Representative results of at least three independent analyses. f Statistical summary of percentage of CD4 + cells in CD8 − mature thymocytes and CD8 − lymph node (LN) T cells of Cd4 ΔE4p/ΔE4p mice and Cd4 ΔE4p/ΔE4p : Bcl11b F/F : Cd4-Cre mice mice. Means ± SD. *** p < 0.001 (unpaired student t test, two-sided). g Dot plots showing CD4 expression and cell divisions five days after in vitro stimulation of sorted CD4 + T cells from mice with indicated genotypes. One representative of three experiments Full size image Considering such Bcl11b associations with Cd4 regulatory regions, we examined Bcl11b function in regulating Cd4 expression by using two Bcl11b mutant models. We recently generated a hypomorphic Bcl11b allele, referred to as Bcl11b m , that produces truncated Bcl11b protein lacking the last zinc-finger domain [23] . In thymi of newborn Bcl11b m/m homozygous mice, which die at two days after birth, CD4 lo CD8 + cells were present in the CD24 hi TCRb lo population, whereas nearly all CD24 hi TCRb lo thymocytes appeared as CD4 + CD8 + DP cells in control mice (Fig. 4c, d ). In addition, CD4 expression in the TCRβ hi CD8 − mature thymocyte population became lower, resulting in the generation of the CD4 − CD8 − instead of CD4 + CD8 − subset in Bcl11b m/m thymi (Fig. 4c, d ). We next examined the effect of conditional inactivation of Bcl11b at DP stage by a Cd4-Cre transgene, and observed emergence of the CD4 − CD8 − subset in the CD24 lo TCRβ hi mature thymocyte population of Bcl11b F/F : Cd4-Cre mice (Fig. 4e ). In order to further address whether Bcl11b regulates E4m activity, we then combined E4p -deficiency with Bcl11b inactivation. Under an E4p -deficient background, the CD4 expression level in the mature CD8-negative thymocyte population severely decreased upon loss of Bcl11b (Fig. 4e, f ). In contrast, CD4 expression level was partially restored after egress from the thymus, with CD4 + T cells emerging in the peripheral lymphoid tissues of Cd4 ΔE4p/ΔE4p : Bcl11b F/F : Cd4-Cre mice (Fig. 4e, f ). However, the CD4 expression in CD4 + T cells that developed in Bcl11b F/F : Cd4-Cre mice were unstable after activation-induced cell divisions (Fig. 4g ). Thus, dysfunction of Bcl11b resulted in a delayed CD4 induction at two transitional stages, one for becoming DP thymocytes and the other for becoming mature CD4 SP thymocytes, which require activation of E4p and E4m , respectively. Characterizing specific activity of E4m In order to further characterize E4m activity, we addressed how E4m alone behaves by generating a Cd4 ΔE4p:ΔS4 allele, in which only the E4m among three regulatory regions remains in the Cd4 gene (Fig. 5a ). Notably, the percentage of cells expressing CD4 was higher in CD8-negative cells than in CD8-positive cells in the mature thymocyte population of Cd4 ΔE4p:ΔS4/ΔE4p:ΔS4 mice (Fig. 5b, c ), although it was equally high in both types of cells of Cd4 ΔS4/ΔS4 mice. To exclude a possibility that deleted sequences around S4 in the Cd4 ΔE4p:ΔS4 allele include a functional element for E4m activity, we targeted specific mutations onto two Runx-motifs within S4 to abrogate S4 function by a more specific manner [9] , generating a Cd4 ΔE4p:S4M allele (Fig. 5a ). In Cd4 ΔE4p:S4M/ΔE4p:S4M mice, the percentage of cells expressing CD4 remained higher in CD8 − cells compared to CD8 + T cells (Fig. 5b, c ). Such CD8 + cells were almost undetected in B2m −/− : Cd4 ΔE4p:S4M/ΔE4p:S4M mice (Supplementary Fig. 4 ), indicating that the majority of CD8 + cells in Cd4 ΔE4p:S4M/ΔE4p:S4M mice constituted MHC-I restricted cells. Given that CD4 expression from the Cd4 ΔE4p:ΔS4 allele is likely to depend on E4m , these observations indicate that the E4m activity is more predominant in the helper-lineage cells than in cytotoxic-lineage cells. Fig. 5 Helper-lineage dominant activity of E4m . a Schematic structures of Cd4 , Cd4 ΔS4 , Cd4 ΔE4p:S4M , and Cd4 ΔE4p:ΔS4 alleles are shown as in Fig. 2a . Mutations at two Runx sites within S4 are marked as X in the Cd4 ΔE4p:S4M allele. b Dot plots showing CD4 and CD8 expression in indicated thymocyte subsets of mice with indicated genotypes. Numbers in quadrants indicate respective cell percentages. Right histograms showing CD4 expression in CD8 + and CD8 − mature (CD24 lo TCRβ hi ) thymocyte populations. Representative results of at least five independent analyses. c Summary of percentage of CD4 + cells in CD8 − and CD8 + mature (CD24 lo TCRβ hi ) thymocyte populations of Cd4 +/+ ( Wt ), Cd4 ΔS4/ΔS4 ( Δ S4 ), Cd4 ΔE4p:S4M/ΔE4p:S4M ( ΔE4p:S4M ), and Cd4 ΔE4p:ΔS4/ΔE4p:ΔS4 (Δ E4p:ΔS4 ) mice. Means ± SD. ** p < 0.01, *** p < 0.001 (unpaired student t test, two-sided) Full size image Regulation of E4m activity by Runx complexes To examine how such helper-lineage dominant activity of E4m is regulated, we analyzed the function of transcription factors that are known to be involved in lineage-specific expression of the Cd4 gene. Two Runx proteins, Runx1 and Runx3, are essential to control lineage specific Cd4 expression through activating the S4 silencer [9] . The penta-peptide sequences, VWRPY, at the C-terminal end of Runx proteins serve as a platform to recruit the TLE/Groucho co-repressor family [24] , [25] , and are essential for Runx-mediated Cd4 repression [10] , [26] . Accordingly, mice lacking the VWRPY motif from both Runx1 and Runx3 proteins ( Runx1/Runx3 ΔV/ΔV mice), exhibited full CD4 de-repression in CD8 + T cells, phenocopying the Cd4 ΔS4/ΔS4 mice (Figs 5b and 6a ). Given a loss of S4 activity by Runx1/Runx3 ΔV/ΔV mutation, we assumed that CD4 expression in Runx1/Runx3 ΔV/ΔV : Cd4 ΔE4p/ΔE4p mice was similar to that in Cd4 ΔE4p:ΔS4/ΔE4p:ΔS4 mice. However, the percentage of CD4-expressing cells was comparable between CD8 + and CD8 − cells in Runx1/Runx3 ΔV/ΔV : Cd4 ΔE4p/ΔE4p mice (Fig. 6a, b ). Thus, a discrepancy existed between the effects from loss of cis -acting S4 and loss of trans- acting Runx proteins on the Cd4 ΔE4p allele, suggesting a possible involvement of S4 -indpendent mechanisms through which Runx proteins suppress E4m activity. We then generated Runx1/Runx3 ΔV/ΔV : Cd4 ΔE4p:S4M/ΔE4p:S4M mice and observed an increase of the CD4 expressing population in CD8 + T cells (Fig. 6a, b ). Our ChIP-qPCR analyses showed that Runx association with the E4m was unaffected by eliminating Runx-motifs in S4 , whereas Runx binding to S4 was abrogated (Fig. 6c ). Together, these observations indicated that Runx proteins are likely to repress E4m activity in a VWRPY-dependent manner through their S4 -independent association with E4m . Fig. 6 Involvement of Runx in regulating the helper-lineage dominant activity of E4m . a Dot plots showing CD4 and CD8 expression in lymph node T cells of mice with indicated genotypes. In Runx1/Runx3 ΔV/ΔV mice, both Runx1 and Runx3 proteins lack the VWRPY motif, which is essential for interaction with TLE/Groucho co-repressors. Right histograms showing CD4 expression level in CD8 − and CD8 + lymph node T cells of Cd4 ΔE4p:S4M/ΔE4p:S4M mice with (lower) or without (upper) Runx1/Runx3 ΔV/ΔV mutation. Numbers in quadrants indicate respective cell percentages. One representative result of three independent analyses. b Summary of percentage of CD4 + cells in CD8 − and CD8 + lymph node T cells of Cd4 ΔE4p/ΔE4p , Cd4 ΔE4p:S4M/ΔE4p:S4M mice with or without Runx1/Runx3 ΔV/ΔV mutation. Means ± SD. ** p < 0.01 (unpaired student t test, two-sided). c Graph showing summary of three independent ChIP-qPCR for Runx bindings to E4p , S4 , and E4m regions in DP thymocytes (DP) and CD8 + T cells from Cd4 +/+ , Cd4 ΔS4/ΔS4 and Cd4 ΔE4p:S4M/ΔE4p:S4M mice. Means ± SD. * p < 0.05, ** p < 0.01 (One-way ANOVA and Tukey’s multiple comparison test) Full size image Lack of canonical Runx-motifs within E4m suggests that recruitment of Runx complexes to E4m might be mediated via protein-protein interaction. As both Bcl11b and Satb1 are functional activators for the E4m enhancer and interact with Runx proteins [23] , [27] , we wished to test whether Runx association with E4m is affected by lack of Bcl11b and Satb1. However, the severe reduction of mature thymocytes in Bcl11b F/F : Satb1 F/F : Cd4-Cre mice (Supplementary Fig. 5a ) made it possible to perform ChIP-qPCR analyses only in DP thymocytes. In this setting, Runx binding to S4 , E4p , and E4m was not significantly changed by the loss of Bcl11b and Satb1proteins (Supplementary Fig. 5b ), suggesting the presence of another factor(s) that recruits Runx complexes to E4m . Repressive regulation of E4m by ThPOK As ThPOK was shown to be essential for the regulation of lineage-specific CD4 expression by counteracting against S4 -mediated Cd4 repression [16] , [28] , we next examined whether ThPOK is involved in the regulation of E4m activity by generating Cd4 ΔE4p:S4M/ΔE4p:S4M :Thpok gfp/gfp mice that lack ThPOK expression. Notably, loss of ThPOK resulted in an increase of CD4 expressing cells in mature CD8 + thymocyte and peripheral CD8 + T cell populations (Fig. 7a, b ). Increase of the CD4 + subset by lack of ThPOK had already been observed at the CD24 hi TCRβ hi stage composed of freshly selected thymocytes and in Thpok-gfp − cells that represent MHC-I-signaled ThPOK non-expressing cells. These genetic results suggested that ThPOK restrains E4m activity from the early initiation phase. Similar early induction of CD4 in CD24 hi TCRβ hi thymocytes from the Cd4 ΔE4p:S4M allele was also observed by Runx1/Runx3 ΔV/ΔV mutation (Fig. 7c ), suggesting that the mechanism by which Runx represses E4m activity became non-functional through the lack of ThPOK expression. Our ChIP-qPCR using peripheral CD4 + T cells showed that ThPOK associated with E4m in the absence of the S4 (Supplementary Fig. 5c ), and Runx association with E4m in pre-selection DP thymocytes was not affected by loss of ThPOK (Fig. 7d ). Interestingly, level of H3K27ac at E4m region tended to be higher in CD8 ± mature thymocytes in the absence of ThPOK, although it was lower than that in control CD4 SP thymocytes ( Supplementary Fig. 5d ) . These observations unraveled an unexpected ThPOK function that assists Runx-mediated repression of E4m activity after recruitment of Runx to the E4m enhancer. Fig. 7 ThPOK is necessary for Runx-mediated repression of E4m activity. a Flow cytometry analyses for CD4, CD8 and Thpok-gfp expression during T cell development in Cd4 ΔE4p:S4M/ΔE4p:S4M mice in the presence or absence of ThPOK. Numbers in quadrants, indicated gate, and the region in histograms indicate respective cell percentages. b Summary of percentage of CD4 + cells in CD8 + mature thymocytes and CD8 + splenic T cells of Cd4 ΔE4p:S4M/ΔE4p:S4M : Thpok +/gfp and Cd4 ΔE4p:S4M/ΔE4p:S4M : Thpok gfp/gfp mice. Means ± SD. *** p < 0.001 (unpaired student t test, two-sided). c Histogram showing CD4 expression in freshly selected (CD24 hi TCRβ hi ) thymocytes of Cd4 ΔE4p:S4M/ΔE4p:S4M : Runx1/Runx3 +/+ and Cd4 ΔE4p:S4M/ΔE4p:S4M : Runx1/Runx3 ΔV/ΔV mice. One representative of two independent analyses. d Graph showing summary of three independent ChIP-qPCR experiments for Runx bindings to E4m in pre-selection DP thymocytes from Cd4 ΔE4p:S4M/ΔE4p:S4M : Thpok +/gfp and Cd4 ΔE4p:S4M/ΔE4p:S4M : Thpok gfp/gfp mice. Means ± SD Full size image By generating several mutant Cd4 alleles, our study provides novel insights into how two enhancers, E4p and E4m , regulate Cd4 expression ( Supplementary Fig. 6 ) . E4p and E4m cooperate to establish a stably heritable active state in the helper-lineage T cells by activating the DNA de-methylation process. It is unclear whether such property is endowed to specific enhancers or is a general feature of enhancers. We showed that a synthetic Eth enhancer derived from the Thpok gene could compensate the E4p activity that induces DNA de-methylation. This suggests that specific sequences within the E4p are unlikely to be absolutely essential to control DNA de-methylation at the Cd4 locus. Despite their differences in sequences, it is possible that Eth and E4p poise similar epigenetic codes that can be recognized by common machinery that induces DNA de-methylation. Recent work reported accumulation of 5hmC, which is generated by TET family proteins through DNA de-methylation processs [29] , near the Thpok proximal enhancer core region in the CD4 SP thymocytes [30] , suggesting that TET proteins are involved in DNA de-methylation for activation of the Thpok gene. Thus, once distinct protein complexes bound on a distinct enhancer marks the target locus with such epigenetic codes, a sequential reaction that induces DNA de-methylation might be carried out. Alternatively, E4p/E4m enhancers and Eth were bound by same nuclear protein(s) that recruit machinery to induce DNA de-methylation. Bcl11b and Satb1 may represent candidates for such shared factors, as both proteins are involved in the activation of E4m in the Cd4 gene and the PE enhancer in the Thpok gene [23] , [27] . This also suggests that activation of the Thpok gene might involve DNA de-methylation. Release of Thpok silencing from CD8 + T cells by an inhibitor for maintenance methyltransferase [31] and the low Thpok expression level effected by a lack of Tet2/3 proteins [15] support the involvement of DNA de-methylation in Thpok activation. In B2m −/− : Cd4 ΔE4m/ΔE4m mice, a re-directed CD4 − CD8 + cell subset is generated in the thymus in part due to impaired ThPOK induction; however, these CD4 − CD8 + thymocytes failed to expand sufficiently to generate a visible population in the periphery. As these cells are MHC-II restricted, the lack of TCR signaling by loss of CD4 expression could impair their survival capacity [32] . However, previous reports have shown that mice expressing a low level of ThPOK retain re-directed CD4 − CD8 + MHC-II restricted cells in the periphery [16] , [33] . It is possible that aberrant CD4 expression kinetics unique to Cd4 ΔE4m/ΔE4m mice may generate CD4 − CD8 + MHC-II restricted cells that acquire IL-7-dependent survival capacity similar to normal MHC-I restricted CD8 SP thymocytes [21] , [22] with a low level of IL-7Ra expression. An imbalance between attaining an IL-7-responsive property and inefficient receptor expression might thus inhibit the expansion of CD4 − CD8 + MHC-II restricted cells in Cd4 ΔE4m/ΔE4m mice. Our genetic results clearly showed that Runx proteins are necessary for S4 -independent repression of E4m activity in CD8 + T cells. Previous research showed that mutant Runt protein, a counterpart of Runx protein in Drosophila , lacking DNA binding activity by point mutations in the Runt-domain, retains the activity to repress the segment polarity gene engrailed ( en ) [34] , indicating that recognition of the Runx-motif is not absolutely necessary for Runx-mediated repression. Once Runx proteins are included into nuclear protein complexes on E4m , TLE/Groucho co-repressor family proteins are likely to be recruited and suppress E4m activity in a CD8-lineage-predominant manner. In contrast, although Runx complexes also associate with the E4p enhancer even in the absence of S4 , inhibition of E4p activity requires S4 sequences. Thus, the modes of Runx action to repress the two enhancers in the Cd4 locus are different, although the VWRPY motif in Runx proteins are shared by two modes. It is possible that protein complexes formed on the S4 region are required specifically to repress transcriptional activators on the E4p enhancer. Alternatively, based on the different position of the two enhancers with respect to S4 , topological regulation such as prevention of chromatin looping between E4p and the P4 promoter may require S4 -dependent regulation. An S4 -independent regulation of lineage specificity of E4m activity challenges the previous silencer-based model that has been proposed to explain how lineage-specific Cd4 expression is regulated. Association of Runx with E4m in both cytotoxic-lineage and helper-lineage cells suggests that Runx-mediated E4m repression is likely to be canceled in a helper-lineage-specific manner. ThPOK was shown to antagonize S4 activity to maintain CD4 expression in helper-lineage cells [16] , [28] . However, our genetic results indicate that ThPOK instead assists Runx-mediated E4m repression. It remains elusive how ThPOK exerts such opposite regulation against S4 -dependent and -independent Runx function. Considering that loss of ThPOK expression affects CD4 expression from the Cd4 ΔE4p:S4M allele in freshly selected thymocytes through MHC-I, it is worth taking into account the possibility that ThPOK expression in early hematopoiesis is involved in later regulation of E4m activity. Recruitment of HDACs was proposed to be a possible mechanism by which ThPOK repress Cd8 gene [19] . Along with a higher H3K27ac status at E4m region in ThPOK-deficient cells, ThPOK might regulate E4m activity via histone acetylation. Alternatively, considering that ThPOK has been shown to be involved in tethering genomic regions to the nuclear lamina to effect gene repression [35] , it is also possible to ThPOK regulate Cd4 expression by altering nuclear positioning of the Cd4 locus during T cell development. Regardless, our genetic results shed new light on the roles of Runx and ThPOK in Cd4 gene regulation by regulating a novel E4m enhancer. Generation of mutant Cd4 alleles In order to generate the target vector for the Cd4 Eth allele, we first generated an Eth DNA fragment by overlap PCR. In the Eth sequences, core enhancer sequences from the thymic enhancer ( TE ) and the proximal enhancer ( PE ) from the Thpok locus were conjugated (Supplementary Fig. 1a ). In order to replace E4p with Eth , the Eth DNA fragment was ligated into the Sal I site of the target vector (a gift from Mark Chong) that was used to generate the E4p Δ/Δ mice [11] . Transfection of target vectors into M1 ES cells and identification of ES clone underwent homologous recombination by PCR were performed. During a process of removal of the neomycin resistant gene (neo r ) by transient transfection of a Cre expression vector, pMC-Cre, ES clones harboring Cd4 +/Eth or Cd4 +/ΔE4p genotype were generated from the into ES clone harboring the Cd4 +/EthN genotype. In order to make the target vector for the Cd4 ΔE4m allele in which mouse genomic region corresponding to 124835251-124835615 in NCBI37/mm9 were deleted (Supplementary Fig. 2b ), we first amplified the 124834833-1283251 region by PCR to add BglII site at 5′ end and SpeI site at 3′ end. In order to make a longer 3′ homology region, a DNA fragment prepared from the pCassette vector [36] by SpeI/KpnI digestion was ligated to the 3′ end. A DNA fragment that harbors 5′ homology region, the neo r gene and the Cd4 silencer region was prepared from the pCassette vector by HindII/BglII digestion, and were ligated together with a BglII/KpnI 3′ homology region into the HindIII/KpnI cleaved pUC18 vector. In order to generate ES clones harboring the Cd4 +/ΔE4m and Cd4 +/ΔE4p:ΔE4m genotype, the target vector for the Cd4 ΔE4m allele was transfected into ES clone harboring Cd4 ΔS4/ΔE4p genotype. After isolating ES clones that underwent homologous recombination, we examined which allele, Cd4 + or Cd4 ΔE4p , was targeted by retroviral Cre transduction, followed by PCR that distinguished pattern of recombination between three loxP sites (Supplementary Fig. 2c ). ES clones harboring the Cd4 +/ΔS4 or Cd4 +/ΔE4p:ΔS4 were similarly generated by transfection of the target vector that remove S4 core region (124835896–124836384 in NCBI37/mm9) into Cd4 +/+ or Cd4 +/Eth ES clone, respectively. ES clones harboring the Cd4 +/ΔE4p:S4M were generated by transfection of the target vector, which was used to target mutation into the Runx sites within the S4 [9] , into the Cd4 +/ΔE4p ES clone. Mice Runx1 ΔV mice [37] , Runx3 ΔV mice [38] , Thpok gfp mice [16] and Bcl11b F and hypomorphic Bcl11b m mice [23] have been described. β2m-deficient mice (002087) were purchased from the Jackson laboratory. Cd4 +/ΔLS mice were generated by crossing Cd4 +/Sflox mice [6] (a gift from Dr. D. R. Littman) to the EIIa-Cre mouse (003724) from the Jackson Laboratory. Generation of chimera mice from ES cells by aggregation was performed by the animal facility at RIKEN, IMS. All mice were maintained in the animal facility at the RIKEN IMS, and all animal procedures were in accordance with protocol approved by the institutional Animal Care and Use Committee (IACUC) of RIKEN Yokohama Branch. Flow cytometry analyses and cell sorting Single cell suspensions from thymus, spleen and lymph nodes were prepared by mashing tissues through a 70 μm cell strainer (BD Bioscience). Single cell suspensions were stained with following antibodies purchased from BD Bioscience or eBiosciences: CD4 (25-0042-81: eBiosciences, RM4-5), CD8α (553035, 563068: BD Biosciences, 53-6.7), CD24 (562563: BD Biosciences, M1/69), CD69 (561931: BD Biosciences, H1.2F3), IL7Rα (17-1271-82: eBiosciences, A7R34) and TCRβ (47-5961-82: eBiosciences, H57-597). For intracellular staining of phosphorylated Stat5 (612599: BD Biosciences, 47), cells were stained with cell surface molecules and were stimulated recombinant mouse IL-7 (R&D) at the indicated time and concentration. After stimulation, cells were fixed and permeabilized with BD Phosflow™ Lyse/Fix buffer (558049: BD Biosciences) and Perm Buffer III (558050: BD Biosciences). Antibodies were used at a concentration of 2.5 μg ml −1 . Multi-color flow cytometry analysis was performed using a BD FACSCanto II (BD-Bioscience) and data were analyzed using FlowJo (Tree Star) software. Cell subsets were sorted using a BD FACSAria II (BD Biosciences). DNA methylation analyses DNA purified from FACS-sorted cells was subjected to bisulfite reactions with MethylEasy™ Xceed (Genetic Signatures) according to the manufacturer’s protocol. PCR product amplified from this DNA was cloned into the pCR TM II Vector using a TA Cloning® Kit (ThermoFisher scientific) and was sequenced. The following primer set was used for PCR amplification: Cd4R1F, 5′-TTGATTTTTTAAAATAGAAAGGTTT-3′ and Cd4R1R, 5′-AAATATCTAAAATATACCAACCACTAC-3′. Quantitative RT-PCR DNase I-treated total RNA was prepared from sorted cells using RNeasy mini kit (QIAGEN) and cDNA was synthesized by SuperScript™ IV reverse transcriptase (ThermoFisher SCIENTIFIC). Quantitative RT-PCR was performed using QuantStudio™ 3 Real-Time PCR system (Applied Biosystems) with Universal ProbeLibrary (Roche). The following primer sets and probes were used for Cd4 and Hprt mRNA quantification: Cd4-F, 5′-TCTGGAACTGCACCGTGAC-3′, Cd4-R, 5′-CCGTGATAGCTGTGCTCTGA-3′ and UPL #93. Hprt-F, 5′-TCCTCCTCAGACCGCTTTT-3′, Hprt-R, 5′-CCTGGTTCATCATCGCTAATC-3′ and UPL #95. Chromatin immune-precipitation (ChIP) ChIP-Seq data for Runx/Cbfβ complexes and Bcl11b binding in total thymocytes were taken from existing deposited data (GEO accession number: GSE90949 and GSE90794, respectively). For analytical ChIP-qPCR, FACS-sorted or MACS (Mitenyi Biotec)-separated 0.5 to 3 × 10 7 cells were used to prepare chromatin DNA. Cells were cross-linked by incubation in a 1% of formaldehyde solution for 10 min with gentle rotation at room temperature. Nuclei were separated and were sonicated using a model XL2000 ultrasonic cell disruptor (MICROSON). Sonicated chromatin was incubated overnight at 4 °C with anti-Histone H3K27ac (clone D5E4, Cell Signaling Technology), anti-Histone H3K27me3 (clone C36B11), 5 ug of anti-Cbfβ rabbit polyclonal antibody [39] , anti-Bcl11b antibody (A300-385A, Bethyl Laboratories) or anti-ThPOK polyclonal antibody [23] that were pre-conjugated with Dynabeads M-280 Sheep anti-Rabbit IgG (Thermo Fisher Scientific). After washing beads, immunoprecipitates were eluted from beads into elution buffer. Eluted immunoprecipitates were then incubated at 65 °C overnight for reverse-crosslinking. Input DNA and ChIP DNA were treated with RNaseA (Thermo Fisher Scientific) and Proteinase K (Thermo Fisher Scientific), and then were purified by ChIP DNA Clean and Concentrator TM kit (ZYMO RESEARCH). Quantitative PCR was performed using the QuantStudio™ 3 Real-Time PCR system (Applied Biosystems) with SYBR Green detection system. 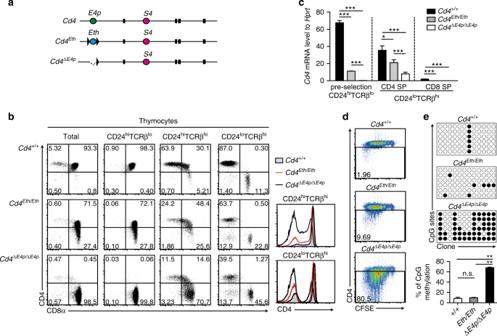Fig. 1 Enhancer replacement betweenCd4andThpokgenes.aSchematic structures of mutantCd4alleles. Ovals marked with different colors represent cis-regulatory regions,Cd4silencer (S4),Cd4proximal enhancer (E4p), and syntheticThpokenhancer (Eth). The black box and triangle represent exons and loxP sequences, respectively.bDot plots showing CD4 and CD8 expression and histograms at the right showing CD4 expression in indicated cell subsets from mice with indicated genotypes. Numbers in quadrants indicate respective cell percentage. Representative results of at least three independent analyses.cGraph showing relativeCd4toHprtmRNA in pre-selection CD24hiTCRβlothymocytes, CD24loTCRβhiCD4 single positive (SP), and CD24loTCRβhiCD8 SP thymocytes of mice with indicated genotypes. Means ± SD. ***p< 0.001, *p< 0.05 ((One-way ANOVA and Tukey’s multiple comparison test)).dPseudocolor plots showing CD4 expression and cell divisions five days after in vitro stimulation of sorted CD4+T cells from mice with indicated genotype. Numbers in the indicated gate represent cell percentages.eBisulfite PCR at six amplicons from the first intron in theCd4gene in naïve CD4+T cells from mice with indicated genotypes. Symbols indicate methylated (black filled circle) or un-methylated (black open circle) CpG motifs. The lower graph shows the summary of three independent experiments. Means ± SD. ***p< 0.01 (unpaired studentttest, two-sided) Primers sequences for quantitative PCR are listed in the Supplementary Table 1 . In vitro T-cell culture Sorted CD4 + T cells were labeled with CFSE (ThermoFisher Scientific) and were cultured in custom ordered Dulbecco’s Modified Eagle Medium (D-MEM, KOHJIN BIO) supplemented with 10% heat inactivated FBS (Hyclone). 2.0 × 10 5 cells were stimulated in 96-well flat-bottomed plate, which was pre-coated with 2 μg ml −1 anti-CD3e antibody (553068, BD Bioscience) and 2 μg ml -1 soluble anti-CD28 antibody (553295, BD Bioscience), for two days, and were maintained in D-MEM supplemented with 10 ng ml -1 recombinant mouse IL-2 (402-ML, R&D system) for 2 to 4 days. Data availability ChIP-seq data that support the findings of this study have been deposited with accession GSE90949 and GSE90794 , respectively. 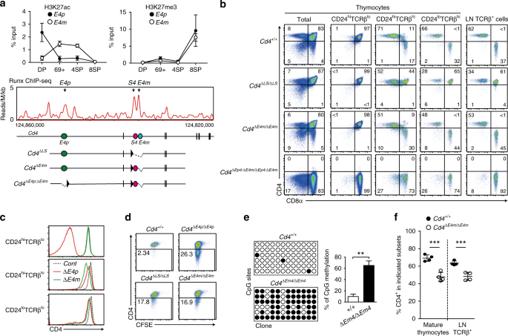Fig. 2 Effects of loss of the maturation enhancer,E4m, on CD4 expression.aUpper graphs showing kinetic changes of H3K27ac and H3K27me3 atE4pandE4mregions in pre-selection (DP), freshly selected (CD69+), and CD4 SP (4SP) and CD8 SP (8SP) thymocytes. Summary of three independent ChIP experiments. Means ± SD. (Middle) Runx ChIP-Seq track at theCd4gene in total thymocytes. Gene structures and regulatory regions are shown as in Fig.1a. Schematic structures of mutantCd4alleles are shown at the bottom.bPseudocolor plots showing CD4 and CD8 expression in indicated cell subsets from mice with indicated genotypes. Numbers in quadrants indicate respective cell percentages. Representative results of at least three independent analyses of each genotype.cHistograms showing CD4 expression levels on CD24hiTCRβlo, CD8-negative CD24hiTCRβhiand CD8-negative CD24loTCRβhithymocytes fromCd4+/+(dotted),Cd4ΔE4p/ΔE4p(red), andCd4ΔE4m/ΔE4m(green) mice. One representative of three analyses.dPseudocolor plots showing CD4 expression and cell divisions five days after in vitro stimulation of sorted peripheral CD4+T cells from mice with indicated genotypes. Numbers in the indicated gate represent cell percentages.eBisulfite PCR analyses of naïve CD4+T cells fromCd4+/+andCd4ΔE4m/ΔE4mmice are shown as in Fig.1d. The right graph shows a summary of three independent experiments. Means ± SD. **p< 0.01 (unpaired studentttest, two-sided).fGraph showing percentage of CD4+CD8−cells in mature (CD24loTCRβhi) thymocytes and the lymph node TCRβ+population ofCd4+/+andCd4ΔE4m/ΔE4mmice. Means ± SD. ***p< 0.001 (unpaired studentttest, two-sided) 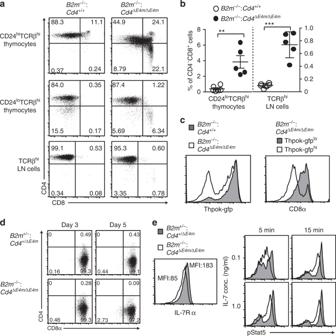Fig. 3 Re-directed differentiation of MHC-II selected thymocyte by loss of theE4menhancer.a,bDot plots inashowing CD4 and CD8 expression in indicated cell subsets fromB2m−/−:Cd4+/+andB2m−/−:Cd4ΔE4m/ΔE4mmice. Graphs inbshowing summary of percentage of CD4−CD8+cells in mature (CD24loTCRβhi) thymocytes and the lymph node (LN) TCRβ+population. Means ± SD. **p< 0.01, ***p< 0.001 (unpaired studentttest, two-sided).cHistogram at left showing Thpok-gfp expression in freshly-selected (CD24hiTCRβhi) thymocytes ofB2m−/−:Cd4+/+andB2m−/−:Cd4ΔE4m/ΔE4mmice. Histogram at right showing CD8 expression in Thpok-gfploand Thpok-gfphiCD24hiTCRβhithymocytes ofB2m−/−:Cd4ΔE4m/ΔE4mmice. One representative result of two mice.dDot plots showing CD4 and CD8 expression three and five days after TCR stimulation of sorted CD4−CD8+mature thymocytes fromB2m+/−:Cd4+/ΔE4mandB2m−/−:Cd4ΔE4m/ΔE4mmice. Numbers in quadrants indicate respective cell percentages.eIL7R expression in CD4−CD8+thymocytes (left) and phosphorylated Stat5 levels in CD4−CD8+thymocytes (right) at 5 and 15 min following IL7 stimulation at indicated concentrations fromB2m+/−:Cd4+/ΔE4mandB2m−/−:Cd4ΔE4m/ΔE4mmice are shown. Numbers in left histograms indicate mean fluorescence intensity (MFI) 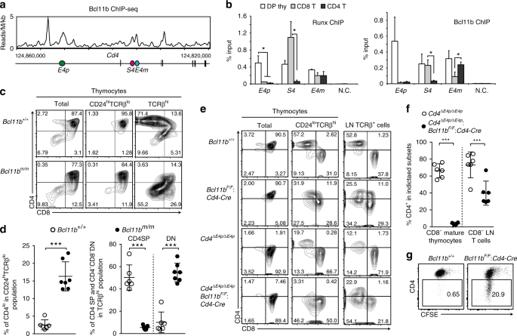Fig. 4 Requirement for Bcl11b in activatingCd4at two stages.aChIP-Seq tracks at theCd4gene showing binding of Bcl11b in total thymocytes.bChIP-qPCR analyses for Runx (left) and Bcl11b (right) bindings to theCd4proximal enhancer (E4p),Cd4silencer (S4), andCd4maturation enhancer (E4m) in DP thymocytes, peripheral CD4+,and CD8+T cells. N.C.: negative control region. Summary of three independent ChIP experiments. Means ± SD. *p< 0.05 (One-way ANOVA and Tukey’s multiple comparison test).cContour plots showing CD4 and CD8 expression in indicated thymocyte subsets ofBcl11b+/+andBcl11bm/mnewborn mice. Numbers in quadrants indicate respective cell percentages. Representative results of at least three independent analyses.dSummary of percentage of indicated cell types in indicated cell populations ofBcl11b+/+andBcl11bm/mmice. Means ± SD. ***p< 0.001 (unpaired studentttest, two-sided).eContour plots showing CD4 and CD8 expression in indicated thymocyte subsets and lymph node (LN) T cells of mice with indicated genotypes. Numbers in quadrants indicate respective cell percentages. Representative results of at least three independent analyses.fStatistical summary of percentage of CD4+cells in CD8−mature thymocytes and CD8−lymph node (LN) T cells ofCd4ΔE4p/ΔE4pmice andCd4ΔE4p/ΔE4p: Bcl11bF/F: Cd4-Cremice mice. Means ± SD. ***p< 0.001 (unpaired studentttest, two-sided).gDot plots showing CD4 expression and cell divisions five days after in vitro stimulation of sorted CD4+T cells from mice with indicated genotypes. One representative of three experiments 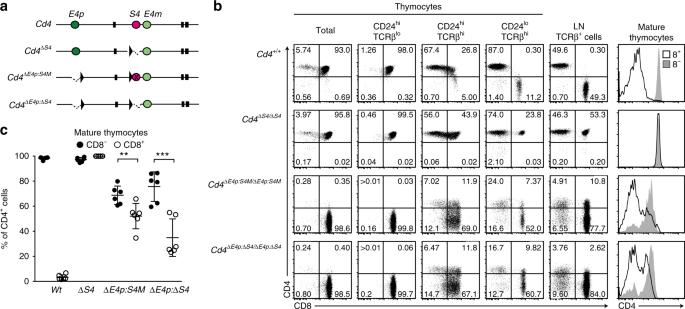Fig. 5 Helper-lineage dominant activity ofE4m.aSchematic structures ofCd4,Cd4ΔS4,Cd4ΔE4p:S4M, andCd4ΔE4p:ΔS4alleles are shown as in Fig.2a. Mutations at two Runx sites withinS4are marked as X in theCd4ΔE4p:S4Mallele.bDot plots showing CD4 and CD8 expression in indicated thymocyte subsets of mice with indicated genotypes. Numbers in quadrants indicate respective cell percentages. Right histograms showing CD4 expression in CD8+and CD8−mature (CD24loTCRβhi) thymocyte populations. Representative results of at least five independent analyses.cSummary of percentage of CD4+cells in CD8−and CD8+mature (CD24loTCRβhi) thymocyte populations ofCd4+/+(Wt),Cd4ΔS4/ΔS4(ΔS4),Cd4ΔE4p:S4M/ΔE4p:S4M(ΔE4p:S4M), andCd4ΔE4p:ΔS4/ΔE4p:ΔS4(ΔE4p:ΔS4) mice. Means ± SD. **p< 0.01, ***p< 0.001 (unpaired studentttest, two-sided) 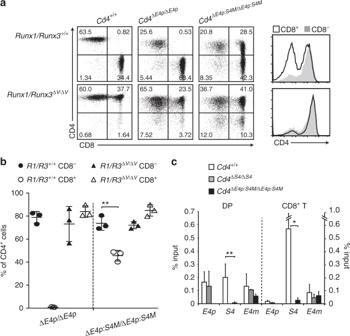Fig. 6 Involvement of Runx in regulating the helper-lineage dominant activity ofE4m.aDot plots showing CD4 and CD8 expression in lymph node T cells of mice with indicated genotypes. InRunx1/Runx3ΔV/ΔVmice, both Runx1 and Runx3 proteins lack the VWRPY motif, which is essential for interaction with TLE/Groucho co-repressors. Right histograms showing CD4 expression level in CD8−and CD8+lymph node T cells ofCd4ΔE4p:S4M/ΔE4p:S4Mmice with (lower) or without (upper)Runx1/Runx3ΔV/ΔVmutation. Numbers in quadrants indicate respective cell percentages. One representative result of three independent analyses.bSummary of percentage of CD4+cells in CD8−and CD8+lymph node T cells ofCd4ΔE4p/ΔE4p,Cd4ΔE4p:S4M/ΔE4p:S4Mmice with or withoutRunx1/Runx3ΔV/ΔVmutation. Means ± SD. **p< 0.01 (unpaired studentttest, two-sided).cGraph showing summary of three independent ChIP-qPCR for Runx bindings toE4p,S4, andE4mregions in DP thymocytes (DP) and CD8+T cells fromCd4+/+,Cd4ΔS4/ΔS4andCd4ΔE4p:S4M/ΔE4p:S4Mmice. Means ± SD. *p< 0.05, **p< 0.01 (One-way ANOVA and Tukey’s multiple comparison test) 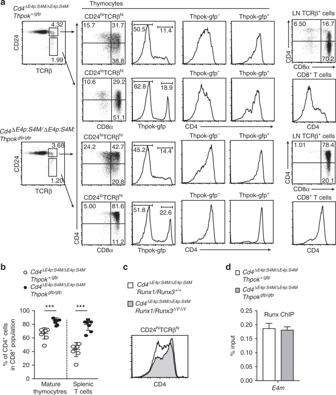Fig. 7 ThPOK is necessary for Runx-mediated repression ofE4mactivity.aFlow cytometry analyses for CD4, CD8 and Thpok-gfp expression during T cell development inCd4ΔE4p:S4M/ΔE4p:S4Mmice in the presence or absence of ThPOK. Numbers in quadrants, indicated gate, and the region in histograms indicate respective cell percentages.bSummary of percentage of CD4+cells in CD8+mature thymocytes and CD8+splenic T cells ofCd4ΔE4p:S4M/ΔE4p:S4M: Thpok+/gfpandCd4ΔE4p:S4M/ΔE4p:S4M: Thpokgfp/gfpmice. Means ± SD. ***p< 0.001 (unpaired studentttest, two-sided).cHistogram showing CD4 expression in freshly selected (CD24hiTCRβhi) thymocytes ofCd4ΔE4p:S4M/ΔE4p:S4M: Runx1/Runx3+/+andCd4ΔE4p:S4M/ΔE4p:S4M: Runx1/Runx3ΔV/ΔVmice. One representative of two independent analyses.dGraph showing summary of three independent ChIP-qPCR experiments for Runx bindings toE4min pre-selection DP thymocytes fromCd4ΔE4p:S4M/ΔE4p:S4M: Thpok+/gfpandCd4ΔE4p:S4M/ΔE4p:S4M: Thpokgfp/gfpmice. Means ± SD All other relevant data are available from the authors.